Transcriptional signature of human pro-inflammatory TH17 cells identifies reducedIL10gene expression in multiple sclerosis We have previously reported the molecular signature of murine pathogenic T H 17 cells that induce experimental autoimmune encephalomyelitis (EAE) in animals. Here we show that human peripheral blood IFN-γ + IL-17 + (T H 1/17) and IFN-γ − IL-17 + (T H 17) CD4 + T cells display distinct transcriptional profiles in high-throughput transcription analyses. Compared to T H 17 cells, T H 1/17 cells have gene signatures with marked similarity to mouse pathogenic T H 17 cells. Assessing 15 representative signature genes in patients with multiple sclerosis, we find that T H 1/17 cells have elevated expression of CXCR3 and reduced expression of IFNG , CCL3 , CLL4 , GZMB , and IL10 compared to healthy controls. Moreover, higher expression of IL10 in T H 17 cells is found in clinically stable vs. active patients. Our results define the molecular signature of human pro-inflammatory T H 17 cells, which can be used to both identify pathogenic T H 17 cells and to measure the effect of treatment on T H 17 cells in human autoimmune diseases. T H 17 cells are a subset of interleukin-17 (IL-17)-secreting T-helper (T H ) cells implicated in the pathogenesis of multiple sclerosis (MS), rheumatoid arthritis, juvenile idiopathic arthritis (JIA), and psoriasis [1] , [2] , whose differentiation is regulated by the transcription factor RAR-related orphan nuclear receptor gamma (RORγt) [3] . Initially, T H 17 cells were considered a uniformly pro-inflammatory population driven by IL-23 and expressed a unique pattern of pro-inflammatory cytokines different from T H 1 and T H 2 cells [4] , [5] , [6] . Subsequent studies showed the function of T H 17 cells in autoimmune diseases and defense against bacterial and fungal pathogens [7] , [8] , [9] , [10] . T H 17 cells can be induced to produce T H 1 and T H 2 cytokines [11] and not all T H 17 cells are pathogenic. Murine T H 17 cells are pathogenic or non-pathogenic based on their ability to induce experimental autoimmune encephalomyelitis (EAE) [12] ; pathogenic T H 17 cells express higher levels of IFN-γ while non-pathogenic T H 17 cells produce IL-10 with IL-17 [13] . As in mice, human T H 17 cells can also co-produce IFN-γ or IL-10. IL-10-producing T H 17 cells are induced in response to Staphylococcus aureus , whereas T H 17 cells induced by Candida albicans produce IL-17 and IFN-γ. Both types of T H 17 cells are enriched in a subset of human memory CD45RA – CD4 + T H cells expressing the chemokine receptors CCR6 and CCR4, while IFN-γ-secreting T H 17 (T H 1/17) cells may additionally express CXCR3 [9] , [14] . A deficiency in IL-17 or the T H 17 pathway compromises host defenses against S. aureus and C. albicans , and reduces the frequency of circulating CCR6 + memory CD4 + T H cells [15] , [16] . Thus both IFN-γ and IL-10-producing T H 17 cells may be protective during infection. IFN-γ and IL-10-producing T H 17 cells are considered pro-inflammatory and anti-inflammatory, respectively, and have opposite functions in autoimmunity [17] , [18] . Studies of T-cell libraries from patients with MS showed that CCR6 + myelin-reactive T cells exhibit enhanced production of IFN-γ, IL-17, and GM-CSF and reduced production of IL-10, when compared with those from healthy individuals [19] . In JIA, IFN-γ-secreting T H 1/17 cells are highly enriched in the synovial fluid (SF) of inflamed joints [20] . The inflammatory environment in diseased joints can induce IFN-γ-negative T H 17 cells to co-produce IFN-γ, implicating plasticity of T H 17 cells [21] . The proportions of T H 1/17-enriched CD4 + CD161 + T cells in the SF of affected joints correlate with the erythrocyte sedimentation rate and serum levels of C-reactive protein, suggesting these cells function in disease pathogenicity [20] . These and other reports of elevated numbers of T H 1/17 cells in inflamed tissues in human autoimmune diseases [21] , [22] , [23] associate T H 1/17 cells with human autoimmune diseases. The complexity of T H 17 function is further manifested in therapeutic studies. Although anti-IL-17 therapy benefits psoriasis, blocking the IL-17 pathway in Crohn’s disease is either ineffective or exacerbates diseases [24] , [25] , [26] . Similarly, in the CD45RB hi adoptive transfer mouse model of experimental colitis, a deficiency of IL-17 production or IL-17R expression in transferred CD45RB hi CD4 T cells results in accelerated disease [27] . The protective function of IL-17 in these studies may be due to the fact that T H 17 cells that line the gut mucosa prevent invasion of the gut microbiome and promote intestinal homeostasis [28] . In tumors, T H 17 cells are reported to have both beneficial [29] , [30] , [31] and detrimental effects [32] both in animal models and human disease. Hence, the function of T H 17 cells in diverse immune responses is complex. We previously reported that murine T H 17 cells can be differentiated into pathogenic vs. non-pathogenic subsets, as well as characterized the molecular signature of murine pathogenic T H 17 cells through global gene expression analysis [12] . In the present study, we compare the gene expression profiles between human IFN-γ + and IFN-γ – T H 17 subsets, and between IL-10 + and IL-10 – T H 17 clones. Comparative transcriptomic analyses show that human T H 1/17 cells and IL-10 – T H 17 clones display gene signatures with marked similarities to mouse pathogenic T H 17 cells. We then assess T H 1/17 cells in patients with MS and find reduced expression of anti-inflammatory IL10 and elevated expression of CXCR3 . When we compare clinically active vs. stable patients, we find that stable patients have higher IL10 expression in T H 17 cells, whereas active patients have higher expression of STAT3 in IFN-γ – /IL-17 – CD4 + T cells. Our results define the molecular signature of human pro-inflammatory T H 17 cells, which can be used to both identify pathogenic T H 17 cells and to measure the effect of treatment on T H 17 cells. Transcriptionally distinct T H 17 subsets in peripheral blood We first performed intracellular cytokine staining of blood CD4 + T cells and identified distinct populations of IFN-γ co-producing T H 17 cells, but no IL-10 co-producing T H 17 cells (Fig. 1a ; Supplementary Fig. 1 ). It is known that IFN-γ + T H 17 cells are increased in inflamed tissues in human autoimmune diseases [21] , [22] , [23] , and are also present in the blood of healthy individuals, whereas IL-10 + T H 17 cells are barely detected [14] . We divided peripheral T H 17 cells into IFN-γ + (T H 1/17) and IFN-γ – (T H 17) subsets. We utilized a capture assay that separates live CD4 + T subsets based on differential secretion of IL-17 and/or IFN-γ to sort ex vivo T H 1/17 cells and T H 17 cells without in vitro polarization and with only short-term (3 h) Phorbol 12-myristate 13-acetate (PMA) plus ionomycin stimulation (Fig. 1b ; Supplementary Fig. 2 ). Based on our global transcriptional analysis of murine T H 17 cells and studies on autoimmunity from ours and other groups, we designed a nanoString nCounter CodeSet HuT H 17 that detects 418 genes associated with human T H cell differentiation and activation. The HuT H 17 CodeSet encompasses genes encoding transcription factors, cytokines, cell surface markers, kinases, lytic proteins, and housekeeping proteins (Supplementary Data 1 ). We used this CodeSet to generate high-throughput transcription profiles of isolated ex vivo T H 1/17, T H 17, T H 1, and double negative (DN) CD4 + T cells from five healthy donors to generate high-throughput transcription profiles. We found high expression of IL17A in T H 17 and T H 1/17 cells and high expression of IFNG in T H 1 and T H 1/17 cells, whereas only minimal expression of IL17A was observed in T H 1 and DN cells and minimal expression of IFNG was observed in T H 17 and DN cells (Fig. 1c ), thus demonstrating that we isolated pure populations of T H 1/17, T H 17, and T H 1 cells. IL10 gene expression was detected in both T H 17 and T H 1/17 cells (Fig. 1d ). Fig. 1 Transcriptionally distinct human T H 17 subsets in peripheral blood. a IFN-γ and IL-10 expression in human T H 17 cells. Isolated PBMCs were stimulated with PMA and ionomycin for 4 h. Production of indicated cytokines in CD4 + T cells were assessed by flow cytometry with intracellular cytokine staining assay. Dotplots shown were gated on CD4 + lymphocytes. Data are representative of two independent experiments with similar results. b Isolation of live T H 1/17, T H 17, T H 1, and DN cells from human PBMC for nCounter analysis. CD4 + T cells isolated from the peripheral blood of healthy donors were stimulated with PMA and ionomycin for 3 h. CD3 + CD4 + -T H 1/17 (IFN-γ + IL-17 + ), T H 17 (IFN-γ − IL-17 + ), T H 1 (IFN-γ + IL-17 − ), and DN (IFN-γ − IL-17 − ) cells were sorted after being stained with fluorescence-conjugated anti-CD3 and CD4 in combination with cytokine secretion detection kits (Miltenyi) ( n = 5). b Isolated CD4 + T subsets were stimulated and stained as in a . c – f CD4 + T-cell subsets treated as in a were measured using the nCounter (nanoString Technologies) CodeSet HuT H 17 and subsequently analyzed (hereafter abbreviated as nCounter analysis). c Differential expression analysis of mRNA levels of IL17A and IFNG . * p < 0.05, ** p < 0.005, *** p < 0.0005, One-way ANOVA with Tukey’s multiple comparison test (mean ± s.d.). d Differential expression analysis of mRNA levels of IL10 . Two tailed, paired Student’s t test p -value was shown (mean ± s.d.). The 326 out of the 418 measured genes in the HuT H 17 CodeSet that showed unsupervised variation across the sample population were used for e hierarchical clustering of the individual samples (individual donors: A, B, C, D, and E), f hierarchical clustering of the Pearson’s linear correlations between the samples (individuals n = 5; individual donors: A, B, C, D, and E), and g principal component analysis of the samples (individuals n = 5) Full size image For the 20 CD4 + T-cell subset samples from the five healthy individuals we analyzed, 362 of the 418 genes demonstrated unbiased variation across the population, defined as an unsupervised expression difference (difference between maximum and minimum relative gene expression values, not taking into account information about the subset classes) ≥5 across all samples, and these genes were selected for further study. Hierarchical clustering of gene expression profiles of the 20 individual samples from the CD4 + subpopulations in the context of these 362 unsupervised varying genes properly segregated the T H 1/17, T H 17, T H 1, and DN cells into four different clusters, revealing their distinct transcriptional features (Fig. 1e ). The in-group Pearson correlation values for these gene expression profiles were high for all four CD4 + T-cell subsets and ranged from 0.95 ± 0.06 for DN cells to 0.98 ± 0.02 for T H 1 cells. Pearson correlation values for the gene expression profiles of T H 1/17 vs. T H 17 and T H 1/17 vs. T H 1 were 0.83 ± 0.05 and 0.78 ± 0.06, respectively, whereas the correlation coefficient for T H 17 vs. T H 1 was only 0.43 ± 0.06 (Fig. 1f ), which were consistent with the degree of similarities observed among the cell subsets in the hierarchical clustering analysis (Fig. 1e ). Principal component analysis (PCA) showed that DN cells were clearly distinct from the other three subsets, whereas T H 1/17 cells lay in between T H 17 and T H 1 cells (Fig. 1g ). These results demonstrate that human T H 17 cells can be transcriptionally categorized into IFN-γ + T H 17 (T H 1/17) and IFN-γ – T H 17 (T H 17) subsets and that T H 1/17 show a close relationship to both T H 17 and T H 1 cells. Human ex vivo T H 17 subsets vs. murine T H 17 cells Murine T H 17 cells generated with TGF-β3/IL-6 or IL-1/IL-6/IL-23 induce more severe EAE than T H 17 cells generated with TGF-β1/IL-6 [12] . In comparing TGF-β3 vs. TGF-β1-induced murine T H 17 cells, we defined a pathogenic transcriptional signature composed of 16 upregulated genes in TGF-β3-induced pathogenic T H 17 cells including CCL3, CCL4, CLL5, CSF2, IL22, IL3, GZMB, STAT4 , and TBX21 [12] . In humans, 10 of the 16 signature genes were upregulated in CCR6 + myelin-reactive memory CD4 + T cells in patients with MS although these cells also displayed elevated levels of IL10 [19] , while 12 genes were upregulated in T H 1/17-enriched CCR7 lo CCR6 + CCR4 lo CXCR3 hi memory CD4 + T cells in healthy donors compared to T H 17-enriched CCR7 lo CCR6 + CCR4 hi CXCR3 lo cells [33] (Supplementary Data 2 ). There are no known unique surface markers for T H 17 cells and all of memory CD4 + T-cell populations contain not only IFN-γ + and IFN-γ – T H 17 cells but also IL-17 – IFN-γ + T H 1 cells, especially for CCR7 lo CCR6 + CCR4 lo CXCR3 hi memory CD4 + T cells, for which the frequency of IL-17 – IFN-γ + cells may be up to four times higher than IL-17 + cells [33] . Among the 14 signature genes shared by murine T H 17 cells and human T H 17-enriched CD4 + T cells, 13 are included in the HuT H 17 CodeSet (Supplementary Data 2 ) and we assessed their expression in T H 1/17, T H 17, T H 1, and DN CD4 + T cells (Fig. 2a ). We found that except for LRMP , the other 12 genes were detected by the CodeSet. Compared to T H 1/17 cells, 10 of the 12 genes had comparable or higher messenger RNA (mRNA) levels in T H 1 cells, which included CCL3, CCL4, CCL5, GZMB, ICOS, IL3, IL7R, LAG3, STAT4 , and TBX21 , emphasizing the importance of minimizing T H 1 contamination when analyzing the gene signature of pro-inflammatory or pathogenic T H 17 cells. The high purity of the T H 1/17 and T H 17 cells we isolated based on IL-17 and IFN-γ secretion allowed us to determine the pathogenicity-associated molecular signature of human T H 17 subsets. Fig. 2 Gene expression comparison between human T H 1/17 vs. T H 17 cells and mouse pathogenic vs. non-pathogenic T H 17 cells. a The expression of previously reported murine and human T H 17 signature genes in purified ex vivo T H 1 cells. The mRNA gene expression levels in T H 1/17, T H 17, T H 1, and DN cells were measured as described in Fig. 1 . * p < 0.05, repeated measures one-way ANOVA; ** p < 0.05, pairwised group comparison with Tukey’s multiple comparison test (mean ± s.d., n = 5). b , c Gene set enrichment analysis comparing human T H 1/17 vs. T H 17 cells with mouse pathogenic vs. non-pathogenic T H 17 cells. b Heatmap of upregulated (upper panels) and downregulated (lower panels) “leading edge” genes of comparison Scenario 1: human T H 1/17 vs. T H 17 cells vs. mouse TGF-β3 plus IL-6-induced T H 17 cells vs. TGF-β1 plus IL-6-induced T H 17 cells (Kolmogorov–Smirnov test p < 0.0001; FDR q < 0.0001 for upregulated genes; Kolmogorov–Smirnov test p = 0.0007; FDR q = 0.001 for downregulated genes). c Heatmap of upregulated (upper panels) and downregulated (lower panels) “leading edge” genes of comparison Scenario 2: human T H 1/17 vs. T H 17 cells vs. mouse IL-1, IL-23 plus IL-6-induced T H 17 cells vs. TGF-β1 plus IL-6-induced T H 17 cells (Kolmogorov–Smirnov test p < 0.0001; FDR q < 0.0001 for upregulated genes; Kolmogorov–Smirnov test p = 0.004; FDR q = 0.004 for downregulated genes). Each column represents one donor in human (n = 5) or one sample in murine ( n = 4). d The robust predicted pathogenic signature (PreP-Signature) of human T H 1/17 cells. Signature genes are those identified as differentially expressed between human T H 1/17 and T H 17 cells that are identified as enriched “leading edge” genes when assessing these human genes in the mouse profiles in b , c and that are additionally curated for robustness based on supervised absolute fold change >1.5. Two tailed, paired Student’s t test p -value < 0.05. * p < 0.05, ** p < 0.05, *** p < 0.0005, n = 5 Full size image We identified 60 genes differentially expressed in T H 1/17 cells vs. T H 17 cells with 39 upregulated and 21 downregulated (Supplementary Data 3 ). To test the hypothesis that the relationship of T H 1/17 to T H 17 cells in humans is similar to that of mouse pathogenic vs. non-pathogenic T H 17 cells, we performed gene set enrichment analysis (GSEA) [34] . The upregulated and downregulated genes in T H 1/17 cells relative to T H 17 cells were divided into two gene sets. Since both TGF-β3/IL-6 and IL-1/IL-6/IL-23 induced mouse pathogenic T H 17 cells whereas TGF-β1/IL-6 induced non-pathogenic T H 17 cells [12] , our first comparison (Scenario I) explored microarray data from TGF-β3/IL-6-induced T H 17 cells (pathogenic) vs. TGF-β1/IL-6-induced T H 17 cells (non-pathogenic) and the second comparison (Scenario II) explored microarray data from IL-1/IL-6/IL-23-induced T H 17 cells (pathogenic) vs. TGF-β1/IL-6-induced T H 17 cells (non-pathogenic). GSEA results demonstrated that genes upregulated in human T H 1/17 vs. T H 17 cells were enriched in mouse pathogenic T H 17 cells vs. non-pathogenic T H 17 cells in both scenarios with 17 “leading edge” genes in Scenario 1 and 19 genes in Scenario 2 (Kolmogorov–Smirnov test p < 0.0001; false discovery rate (FDR) q < 0.0001 for both scenarios) (upper panels of Fig. 2b, c ). The “leading edge” subset of genes is defined as genes that drive the enrichment scores, thus the genes that appear in the top of the ranked list of genes at, or before, the point where the running sum reaches the maximum deviation from zero. The “leading edge” subset can be interpreted as the core subset of a gene set that accounts for the enrichment signal [34] . Genes upregulated in human T H 17 vs. T H 1/17 cells were also enriched in mouse non-pathogenic T H 17 cells vs. pathogenic T H 17 cells in both comparison scenarios, with seven identical “leading edge” genes (Kolmogorov–Smirnov test p = 0.0007; FDR q = 0.001 for Scenario I; Kolmogorov–Smirnov test p = 0.004; FDR q = 0.004 for Scenario II) (lower panels of Fig. 2b, c ). The gene signatures obtained from both scenarios were almost identical even though the TGF-β3/IL-6-induced T H 17 cells and IL-1/IL-6/IL-23-induced T H 17 cells were differentiated via treating naive CD4 + T cells with different cytokines, suggesting that the integrated gene expression analysis identified common features shared by the two types of mouse pathogenic T H 17 cells. Thus, we found marked similarities in differential gene expression signatures between human IFN-γ + vs. IFN-γ – T H 17 cells and mouse pathogenic vs. non-pathogenic T H 17 cells indicating that human T H 1/17 and T H 17 cells are counterparts of murine pathogenic and non-pathogenic T H 17 cells. Among the 27 signature genes identified in both comparison scenarios, 13 had an absolute fold change >1.5 for T H 1/17 vs. T H 17 cells, which were selected as the robust predicted pathogenic signature (PreP-Signature) of T H 1/17 cells for later analyses (Fig. 2d ). The upregulated robust PreP-Signature genes with pro-inflammatory/pathogenic potential can be grouped into chemokines and cytokines ( CCL3 , CCL4 , CCL5 , CSF2 , IFNG , and IL3 ), chemokine and cytokine receptors ( CXCR3 and IL23R ), cytokine responding genes ( EPSTI1 ), effector proteins ( GZMB ), and signaling molecules ( RGS2 ). The downregulated genes are the chemokine receptor ( CCR6 ) and the transcription factor ( STAT1 ). We also investigated genes not shared between human and mouse pathogenic/non-pathogenic Th17 cells to identify other potentially relevant genes to test in human conditions. We identified 33 non-shared genes including 19 that were upregulated and 14 that were downregulated (Supplementary Data 4 ). Human ex vivo T H 17 subsets vs. T H 17 clones IL-10 has a pivotal role in regulation of both innate and adaptive immunity [35] and murine TGF-β1/IL-6-induced non-pathogenic T H 17 cells produce IL-10 [13] . Human IL-10 + T H 17 cells are a potential counterpart of mouse non-pathogenic T H 17 cells. However, IL-10-secreting T H 17 cells cannot be directly isolated from human blood for nCounter gene expression analysis because few or no T H 17 cells produce IL-10 after PMA/ionomycin stimulation (Fig. 1a ). This is likely due to the delayed production of IL-10 after stimulation. Nonetheless, for established human T H 17 clones, IL-10 + T H 17 clones can be identified by IL-10 intracellular staining 5 days after T-cell receptor activation [9] . Thus, we established CD4 + T cells clones from CCR6 + CCR4 + CXCR3 – memory CD4 + T cells (Supplementary Fig. 3 ) that were enriched for T H 17 cells [14] , [18] and screened for clones producing IL-17 with or without co-secretion of IL-10. qRT-PCR showed that IL-10 – T H 17 clones expressed high levels of IFNG , low levels of IL10 , and high levels of IL23R , whereas IL-10 + T H 17 clones expressed minimal levels of IFNG and high levels of IL10 (Fig. 3a ). To assess whether the gene expression profile of cloned T H 17 cells maintained their pro or anti-inflammatory features after long-term culture, we used the HuT H 17 CodeSet to analyze the gene expression profile of IL-10 – and IL-10 + T H 17 clones. We identified 63 genes that were differentially expressed between IL-10 – vs. IL-10 + T H 17 clones with 49 upregulated and 14 downregulated genes (Supplementary Data 5 ). To compare genes differentially expressed between human T H 1/17 vs. T H 17 cells (Supplementary Data 3 ) to those between IL-10 – vs. IL-10 + T H 17 clones (Supplementary Data 5 ), we assessed enrichment of overlaps between gene lists using the hypergeometric enrichment test. We found that genes upregulated in T H 1/17 vs. T H 17 cells display significant overlap with genes upregulated in IL-10 – vs. IL-10 + T H 17 clones (one-sided Fisher’s exact test p < 0.0001, FDR q = 0.0001) (Fig. 3b ). The upregulation of CBLB, CLL5, CXCR3, IL23R, REL, TBX21 , and TNFSF14 in IL-10 – T H 17 clones is shared by human T H 1/17 cells and mouse pathogenic T H 17 cells (Fig. 2b, c ). To identify regulatory molecules predicted to influence the differentiation/development of T H 1/17 cells and IL-10 – T H 17 clones, we interrogated genes differentially expressed between T H 1/17 vs. T H 17 cells (Supplementary Data 3 ) and between IL-10 – vs. IL-10 + T H 17 clones (Supplementary Data 5 ) for upstream regulator prediction analysis in ingenuity pathway analysis (IPA). T H 1/17 cells and IL-10 – T H 17 clones displayed a similar pattern of the activation of signaling pathways involved in T H 17 differentiation/development (Fig. 3c ), especially for activation of IL-1β signaling, which is critical to promote co-producing IFN-γ and to inhibit IL-10 production in T H 17 cells [9] . These results demonstrate the similarities between T H 1/17 vs. T H 17 cells and IL-10 – vs. IL-10 + T H 17 clones, and also indicate that IL-10 – and IL-10 + T H 17 clones maintained their pro- or anti-inflammatory characteristics after long-term culture. Fig. 3 Gene expression comparison between human T H 1/17 vs. T H 17 cells and IL-10 – vs. IL-10 + T H 17 clones. a Quantitative RT-PCR analysis of gene expression in human IL-10 – and IL-10 + T H 17 clones isolated from healthy donors (two tailed, paired Student’s t test, mean ± s.d., n = 3). For IFNG , IL17A , and IL23R , resting T H 17 clones were stimulated with anti-CD3 and anti-CD28 for 4 h before RNA extraction. For IL10 , resting T H 17 clones were stimulated with anti-CD3 and anti-CD28 for 5 days, then cells were re-stimulated with anti-CD3 and anti-CD28 for 4 h before RNA extraction. b Hypergeometric enrichment test between human T H 1/17 vs. T H 17 cells and IL-10 – vs. IL-10 + T H 17 clones. Genes differentially expressed between human T H 1/17 and T H 17 cells (Supplementary Data 3 ) were analyzed for enrichment in those of human IL-10 – vs. IL-10 + T H 17 clones (Supplementary Data 5 ). Heatmap shows the overlapping genes (one-sided Fisher’s exact test p < 0.0001, FDR q = 0.0001). Each column represents one donor ( n = 5). c Predicted upstream regulators for T H 1/17 and IL-10 – T H 17 clone differentiation. The differentially expressed genes with corresponding fold changes and p -values from the T H 1/17 vs. T H 17 comparison (Supplementary Data 3 ) and IL-10 – vs. IL-10 + T H 17 clone comparison (Supplementary Data 5 ) were analyzed using the IPA upstream regulator analysis. Ex vivo, T H 1/17 vs. T H 17 comparison; Clone, IL-10 – vs. IL-10 + T H 17 clone comparison. d , e Gene set enrichment analysis comparing human IL-10 – vs. IL-10 + T H 17 clones with mouse pathogenic vs. non-pathogenic T H 17 cells. d Heatmap of upregulated (upper panels) and downregulated (lower panels) “leading edge” genes of comparison Scenario 1: human IL-10 – vs. IL-10 + T H 17 clones vs. mouse TGF-β3 plus IL-6-induced T H 17 cells vs. TGF-β1 plus IL-6-induced T H 17 cells (Kolmogorov–Smirnov test p = 0.004; FDR q = 0.005 for upregulated genes; Kolmogorov–Smirnov test p = 0.004; FDR q = 0.003 for downregulated genes). e Heatmap of upregulated (upper panels) and downregulated (lower panels) ‘‘leading edge” genes of comparison Scenario 2: human IL-10 – vs. IL-10 + T H 17 clones vs. mouse IL-1, IL-23 plus IL-6-induced T H 17 cells vs. TGF-β1 plus IL-6-induced T H 17 cells (Kolmogorov–Smirnov test p = 0.005; FDR q = 0.010 for upregulated genes; Kolmogorov–Smirnov test p = 0.016; FDR q = 0.009 for downregulated genes). Each column represents one donor in human ( n = 5) or one sample in murine ( n = 4) Full size image Human T H 17 clones vs. murine T H 17 cells We performed GSEA to investigate the similarity between human T H 17 clones and mouse T H 17 cells. The upregulated and downregulated genes in IL-10 – T H 17 clones relative to IL-10 + T H 17 clones T H 17 cells were divided into two gene sets (Supplementary Data 5 ) to explore the enrichment of the gene sets in Scenarios I and II (defined above). GSEA showed that genes upregulated in IL-10 – vs. IL-10 + T H 17 clones were enriched in mouse pathogenic vs. non-pathogenic T H 17 cells in both scenarios, with 17 “leading edge” genes in Scenario I (Kolmogorov–Smirnov test p = 0.004; FDR q = 0.005) and 14 “leading edge” genes in Scenario II (Kolmogorov–Smirnov test p = 0.005; FDR q = 0.010). Among the “leading edge” genes, 11 overlapped between both scenarios (upper panels of Fig. 3d, e ). Genes upregulated in human IL-10 + vs. IL-10 – T H 17 clones were also enriched in mouse non-pathogenic vs. pathogenic T H 17 cells in both scenarios, with six “leading edge” genes in Scenario I (Kolmogorov–Smirnov test p = 0.004; FDR q = 0.003) and seven “leading edge” genes in Scenario II (Kolmogorov–Smirnov test p = 0.016; FDR q = 0.009). Among the “leading edge” genes, six genes were represented in both scenarios (lower panels of Fig. 3d, e ). These results demonstrate extensive similarities between human IL-10 – vs. IL-10 + T H 17 clones and mouse pathogenic vs. non-pathogenic T H 17 cells. T H 17 PreP-signatures predict STAT3 as an upstream regulator Integrated analysis of gene expression profiles of human ex vivo T H 17 cells, human T H 17 clones, and cytokine-induced mouse T H 17 cells resulted in four sets of gene signatures associated with the pathogenicity of T H 17 cells (Figs. 2 , 3 ). We merged the “leading edge” genes from the above GSEA comparisons and consolidated these four gene signatures into one complete PreP-Signature for human ex vivo T H 17 cells with 27 signature genes and one complete PreP-Signature for human T H 17 clones with 26 signature genes. Among the signature genes upregulated in human T H 1/17 cells and IL-10 – T H 17 clones, seven genes were shared by both types of T H 17 cells, while for downregulated genes, two genes overlapped between T H 1/17 cells and IL-10 – T H 17 clones (Fig. 4a ). Since our molecular signatures derive from integrated analysis of pro-inflammatory human T H 17 cells with mouse pathogenic T H 17 cells in autoimmunity, they reduce the number of potential targeting genes and also help define human T H 17 cells with potential pathogenicity in autoimmunity. Fig. 4 Predicting STAT3 as upstream transcription factor by the PreP-Signatures of T H 17 cells. a Venn diagram representations of signature genes upregulated (left) and downregulated (right) in human T H 1/17 cells and IL-10 – T H 17 clones. Complete PreP-Signatures from GSEA comparison Scenarios I and II were merged for ex vivo cells (Fig. 2b, c ) and T H 17 clones (Fig. 3d, e ), respectively. Genes with supervised absolute fold change >1.5 in either ex vivo cells or T H 17 clones were shown in italic bold letters. Ex vivo, differentially expressed “leading edge” genes from T H 1/17 vs. T H 17 GSEA comparisons presented in green circles; Clone, differentially expressed “leading edge” genes from IL-10 – vs. IL-10 + T H 17 clone GSEA comparisons presented in yellow circles. b Predicted upstream transcription factors for T H 1/17 and IL-10 – T H 17 clone differentiation. The molecular signatures of T H 1/17 cells and IL-10 – T H 17 clones in a were analyzed using the Enrichr ChEA2016 analysis and the predicted transcription factors with Benjamini–Hochberg adjusted p -value <0.05 were shown. TF transcription factor Full size image We interrogated the complete PreP-Signatures of ex vivo T H 1/17 cells and IL-10 – T H 17 clones for upstream transcription factor prediction analysis using the Enrichr ChEA2016 analysis [36] , [37] . STAT3 in CD4 + T cells was the top predicted transcription factor common for both resulting lists (Fig. 4b ; Supplementary Datas 6 , 7 ) and thus may regulate the pathogenicity of human T H 17 cells in autoimmune diseases. 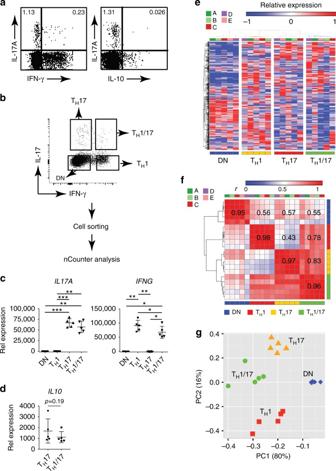Fig. 1 Transcriptionally distinct human TH17 subsets in peripheral blood.aIFN-γ and IL-10 expression in human TH17 cells. Isolated PBMCs were stimulated with PMA and ionomycin for 4 h. Production of indicated cytokines in CD4+T cells were assessed by flow cytometry with intracellular cytokine staining assay. Dotplots shown were gated on CD4+lymphocytes. Data are representative of two independent experiments with similar results.bIsolation of live TH1/17, TH17, TH1, and DN cells from human PBMC for nCounter analysis. CD4+T cells isolated from the peripheral blood of healthy donors were stimulated with PMA and ionomycin for 3 h. CD3+CD4+-TH1/17 (IFN-γ+IL-17+), TH17 (IFN-γ−IL-17+), TH1 (IFN-γ+IL-17−), and DN (IFN-γ−IL-17−) cells were sorted after being stained with fluorescence-conjugated anti-CD3 and CD4 in combination with cytokine secretion detection kits (Miltenyi) (n= 5).bIsolated CD4+T subsets were stimulated and stained as ina.c–fCD4+T-cell subsets treated as inawere measured using the nCounter (nanoString Technologies) CodeSet HuTH17 and subsequently analyzed (hereafter abbreviated as nCounter analysis).cDifferential expression analysis of mRNA levels ofIL17AandIFNG. *p< 0.05, **p< 0.005, ***p< 0.0005, One-way ANOVA with Tukey’s multiple comparison test (mean ± s.d.).dDifferential expression analysis of mRNA levels ofIL10. Two tailed, paired Student’sttestp-value was shown (mean ± s.d.). The 326 out of the 418 measured genes in the HuTH17 CodeSet that showed unsupervised variation across the sample population were used forehierarchical clustering of the individual samples (individual donors: A, B, C, D, and E),fhierarchical clustering of the Pearson’s linear correlations between the samples (individualsn= 5; individual donors: A, B, C, D, and E), andgprincipal component analysis of the samples (individualsn= 5) Investigation of PreP-Signature genes in multiple sclerosis To investigate PreP-Signature genes in human pro-inflammatory T H 17 cells in MS, we isolated T H 1/17 and T H 17 cells from untreated patients with relapse-remitting MS (RRMS) and age and sex-matched healthy controls (Table 1 ; Supplementary Fig. 2 ), assessed frequencies of T H 1/17 and T H 17 cells, and measured the expression of the PreP-Signature genes. T H 1 and DN cells were isolated in parallel as internal controls. Of 19 patients with RRMS, sufficient RNA for quantitative PCR (qPCR) analysis was obtained from 15 T H 1/17 samples, 18 T H 17 samples, 19 T H 1 samples, and 19 DN samples. Of 16 healthy controls, we obtained sufficient RNA for qPCR analysis from 16 T H 1/17 samples, 14 T H 17 samples, 16 T H 1 samples, and 16 DN samples. We found no difference in frequency of T H 1/17, T H 17, and total T H 17 cells among total CD4 + T cells in patients vs. controls (Fig. 5a ). The percentage of T H 1/17 in total T H 17 cells was also similar (Fig. 5b ). To assess purity of isolated cell subsets, we measured the expression of IL17 and IFNG by qPCR. We detected high levels of IL17 in T H 1/17 and T H 17 cells but not in DN cells (Supplementary Fig. 4a ), and high levels of IFNG in T H 1/17 cells but not in T H 17 and DN cells (Supplementary Fig. 4b ), demonstrating that the isolated populations were of high purity. In both groups, IL17 expression was higher in T H 17 vs. T H 1/17 cells (Supplementary Fig. 4a ), whereas IL17 expression was similar for T H 1/17 and T H 17 cells (Fig. 5c ). To validate the 13 robust PreP-Signature genes identified via the nCounter analysis, we measured their expression in T H 1/17 and T H 17 cells in healthy controls by qPCR (Fig. 5d , left). For the 11 genes upregulated in T H 1/17 cells, 9 were confirmed; the 2 downregulated genes were not validated. In MS, the nine validated genes displayed the similar upregulated expression pattern (Fig. 5d , right). Thus, the transcriptional regulation of the nine validated robust PreP-Signature genes of T H 1/17 cells was tightly associated with IFN-γ secretion in both controls and MS. These results indicate that studying frequency or number of IFN-γ-secreting T H 17 cells may not identify important biological differences. Table 1 Demographics of patients with multiple sclerosis and healthy controls Full size table Fig. 5 Frequency of T H 17 subsets and differential expression of PreP-Signature genes in T H 1/17 vs. T H 17 cells in MS. Peripheral CD4 + T cells isolated from the PBMC of untreated RRMS patients ( n = 19) and age- and sex-matched healthy controls (HC) ( n = 16) were stimulated, stained, and sorted for T H 1/17, T H 17, T H 1, and DN cells as described in Fig. 2b . RNA isolated from sorted cell subsets was subjected to low-input qPCR analysis. a Frequencies of T H 1/17, T H 17, and total T H 17 cells in total peripheral CD4 + T cells (Welch’s t test, p -values, mean ± s.d.). b Frequency of T H 1/17 in total T H 17 cells (Welch’s t test, mean ± s.d.). c , d qPCR analysis of gene expression in isolated CD4 + T-cell subsets. c Comparison of IL17A expression between HC and patients in T H 1/17 or T H 17 cells (Welch’s t test, mean ± s.d.). d Differential expression of PreP-Signature genes between T H 1/17 vs. T H 17 cells in HC and MS patients. Two tailed, paired Student’s t test, * p < 0.05, ** p < 0.001, *** p < 0.0001 Full size image We investigated differences between MS and control using the robust PreP signature genes we identified above. We first measured the expression of the 13 robust PreP-Signature genes in T H 1/17 cells in MS and found elevated expression of CXCR3 and reduced expression of IFNG , CCL3 , CLL4 , and GZMB (Fig. 6a ). In T H 17 cells, GZMB showed reduced expression in MS (Fig. 6b ). No difference was observed between MS and controls in T H 1 cells (Supplementary Fig. 5 ). Thus, the altered expression of these five PreP-Signature genes are specific for T H 1/17 and T H 17 subsets, but not for T H 1 cells. We then measured the expression of TBX21 and IL10 , since we found downregulation of TBX21 and upregulation of IL10 in IL-10 + T H 17 clones (Fig. 3a, d ). We found TBX21 expression elevated in T H 1/17 relative to T H 17 cells in MS and controls (Fig. 6c , upper panel), with no difference in IL10 expression (Fig. 6d , upper panel). However, when we compared T H 1/17 and T H 17 cells between MS and controls, IL10 was reduced in T H 1/17 and T H 17 cells in patients (Fig. 6d , lower panel), though no difference was detected with TBX21 expression (Fig. 6c , lower panel). The predicted upstream transcription factor STAT3 was elevated in the DN cells in MS (Fig. 6e , upper panel), while the expression of its antagonistic transcription factor STAT5A [38] , [39] , [40] was reduced (Fig. 6e , lower panel). Fig. 6 Expression of PreP-signature genes of human pro-inflammatory T H 17 cells in RRMS. RNA isolated from T H 1/17, T H 17, and DN cells (Fig. 5 ) was subjected to qPCR analysis. Comparison of PreP-Signature gene expression between HC and patients with RRMS in a T H 1/17 cells and b T H 17 cells. (Welch’s t test, mean ± s.d.). Comparison of c TBX21 and d IL10 expression between HC and patients with RRMS in T H 1/17 and T H 17 cells. e Comparison of STAT3 (upper panel) and STAT5A (lower panel) expression between HC and patients with RRMS in T H 1/17, T H 17, and DN cells. Welch’s t test p -values were shown (mean ± s.d.) Full size image Thus, the altered expression of five PreP-Signature genes for T H 1/17 cells in MS ( CXCR3 , IFNG , CCL3 , CLL4 , and GZMB ) is T H 17-specific. The low expression of IL10 in CXCR3 hi T H 1/17 cells in MS suggests these pro-inflammatory cells may more readily migrate to central nervous system (CNS) since CXCL10 (IP-10), a ligand for CXCR3, is increased in the inflamed CNS in MS [41] , [42] , [43] , [44] . It has been suggested that STAT3 facilitates T H 17 differentiation and STAT5 facilitates Treg differentiation [38] , [39] , [40] , which is consistent with our observation of their expression in DN cells in MS. We then investigated whether the PreP-Signature genes, which had altered expression in MS, were linked to disease activity in MS. Disease activity was defined as a gadolinium-enhancing lesion on magnetic resonance imaging (MRI) or disease relapse within 6 months to the time of blood sampling. All patients were untreated at the time of blood sampling. From 12 active patients, we obtained sufficient RNA for qPCR from 8 T H 1/17 samples, 12 T H 17 samples, and 12 DN samples. From seven stable patients, we obtained sufficient RNA for qPCR from 7 T H 1/17 samples, 6 T H 17 samples, and 7 DN samples. We found reduced expression of IL10 in T H 17 cells (primarily in T H 1/17 cells) and increased expression of STAT3 in DN cells in active patients with RRMS (Fig. 7 ). Given the facilitating role of STAT3 in T H 17 differentiation and the anti-inflammatory function of IL-10, these results together with the altered expression of CXCR3 , IFNG , CCL3 , CLL4, GZMB , IL10 , STAT3 , and STAT5A in MS (Fig. 6 ) are consistent with an important role for T H 17 cells in MS. Fig. 7 Correlation of IL10 and STAT3 expression with disease activity in MS. The mRNA levels of signature genes with altered expression in MS (Fig. 6 ) were compared between active and stable patients. Signature gene expression in a T H 1/17 (active, n = 8; stable, n = 7), b T H 17 (active, n = 12; stable, n = 6), and c DN cells (active, n = 12; stable, n = 7) (Welch’s t test, mean ± s.d.) Full size image We found human IL-17-secreting CD4 + helper T cells were distinct from T H 1 cells, and could be transcriptionally segregated into IFN-γ + T H 17 (T H 1/17) and IFN-γ – T H 17 (T H 17) subsets. On a transcriptional level, T H 1/17 cells have features of both T H 17 and T H 1 cells. In addition to IFN-γ, T H 1/17 cells expressed elevated levels of the pro-inflammatory molecules CCL3, CCL4, CCL5, granzyme B, IL-3, IL-22, GM-CSF, STAT1, T-bet, and IL-23R, which are pathogenic signature genes of mouse T H 17 cells [12] . These results not only transcriptionally segregate human T H 1/17 cells from other T H 17 cells, but also indicate that these cells have acquired pro-inflammatory properties similar to murine pathogenic T H 17 cells. This provided the foundation for the cross-species comparative transcriptomic analysis between mouse and human. We compared the gene expression profiles of human T H 1/17 cells vs. T H 17 cells with mouse pathogenic vs. non-pathogenic T H 17 cells via GSEA and found human T H 1/17 vs. T H 17 cells displayed gene expression signatures that were enriched in mouse pathogenic vs. non-pathogenic T H 17 cells. We obtained similar results in comparing human IL-10 – vs. IL-10 + T H 17 clones with and mouse pathogenic vs. non-pathogenic T H 17 cells. Through this integrated analysis, we identified gene expression features to support the hypothesis that T H 1/17 cells are the pathogenic T H 17 population in immune-mediated human disease. The PreP-Signature genes derived from comparative transcriptional analysis of human and mouse studies identify genes shared between human T H 1/17 vs. T H 17 cells or between human IL-10 – vs. IL-10 + T H 17 clones and mouse pathogenic vs. non-pathogenic T H 17 cells. We obtained a robust PreP-Signature for T H 1/17 cells of 13 genes and assessed them in MS. We find that T H 1/17 cells in patients with MS have elevated expression of CXCR3 and reduced expression of IL10 . It has been shown that CXCL10 (IP-10), a ligand for CXCR3, is increased in the inflamed CNS of MS [41] , [42] , [43] , [44] . Given that IL-10 is a potent anti-inflammatory cytokine, this combination may facilitate migration of more pro-inflammatory CXCR3 hi IL-10 low T H 1/17 cells to the inflamed CNS. However, it is unexpected to observe reduced expression of signature genes IFNG , CCL3 , CLL4 , and GZMB in T H 1/17 cells in MS vs. healthy controls, especially the reduced expression of IFNG . Natalizumab, a humanized monoclonal antibody targeting α4 integrin used in the treatment of MS, functions by preventing immune cells from crossing the blood–brain barrier [45] . A study has shown that both natalizumab treated and untreated patients during relapse have lower frequencies of T H 17 cells in peripheral blood compared to stable patients. Moreover, T H 17 cells become almost undetectable in patients with breakthrough disease that occurs following natalizumab withdrawal [46] . Thus, one explanation for reduced expression of IFNG , CCL3 , CLL4 , and GZMB in T H 1/17 cells in MS could be that migration of cells to the CNS removes CXCR3 high, active T H 1/17 cells from the blood. Another possibility may be that expression of IFN-γ ensures high expression of CXCR3, which is critical for cells to migrate to inflamed CNS, and reduced IFN-γ may indicate the further enhancement of the pathogenicity of IL-10 lo T H 17 cells in MS. IFN-γ-stimulation is required for CXCR3 induction on T cells upon T-cell receptor stimulation [47] . Although counter-intuitive, the potent pro-inflammatory T H 1 cytokine IFN-γ is protective during EAE induction [48] , [49] , [50] . It suppresses EAE induction by inhibiting generation of T H 17 cells [51] , converting CD4 + CD25 – T cells to CD4 + Tregs [52] and limiting myelin lipid peroxidation in CNS [53] . IFN-γ is dispensable for generation of pathogenic T H 17 cells, however, T-bet the transcription factor for T H 1 was initially considered essential due to the high resistance of Tbet −/− mice to EAE [54] , [55] . Later studies show that T-bet is essential for T H 1 but not T H 17-mediated EAE [56] , [57] . Studies in Tbet −/− mice have shown that reduced IFN-γ in T H 17 cells does not affect their pathogenicity though the conversion of T H 17 cells to T H 1/17 cells as well as T H 1-like IFN-γ + ex-T H 17 cells is prevented [56] , [58] , [59] . Interrogating the PreP-Signatures for the identification of upstream regulators and transcription factors [36] , [37] , we identified STAT3 as the top predicted upstream transcription factor from previous studies in CD4 + T cells, which suggests that STAT3 may regulate the pathogenesis of human T H 17 cells in autoimmune diseases. It has been reported that STAT3 is a critical regulator for the induction of T H 17 cells in humans. Humans with a genetic defect in STAT3 expression not only have reduced expression of T H 17 without any impact on other T-cell subsets, but also develop a hyper-IgE syndrome with severe infections of C. albicans and S. aureus [60] , [61] . STAT3 and STAT5 are a pair of mutual restraint transcription factors that regulate T H 17 and Treg differentiation with STAT3 facilitates T H 17 differentiation and STAT5 facilitates Treg differentiation [38] , [39] , [40] . We thus investigated the expression of STAT3 and STAT5A in MS. We found upregulation of STAT3 and downregulation of STAT5A in DN cells from patients with MS, which included naive and other memory CD4 + T cells but not T H 1/17, T H 17, and T H 1 cells. One explanation for the different behavior of STAT3 and STAT5A between DN vs. T H 1/17 and T H 17 cells is that STAT3 may be critical for T H 17 differentiation but not required for T H 17-associated immunopathology after differentiation. Leveraging comparative transcriptomic approaches, we integrated gene expression profiles derived from human and mouse T H 17 cells to identify pathogenicity-associated signature (PreP-Signature) genes that are shared by human pro-inflammatory T H 17 cells and mouse pathogenic T H 17 cells, and to predict the upstream regulators or transcription factors that may be critical for the differentiation of human pro-inflammatory T H 17 cells. These comparative transcriptomic analyses allowed us to identify altered gene expression associated with T H 17 subsets and their differentiation in subjects with MS and to identify associations of the expression of STAT3 in DN cells and IL10 in T H 17 cells that are dependent on MS disease activity. Of note, we used a nCounter codeset with a limited set of pre-selected 418 genes, which may miss other disease related, highly discriminant genes in humans. Thus, follow-up studies, such as RNA-sequencing analysis on T H 17 and T H 1/17 subsets isolated from MS patients, may help to identify more disease-related genes. In summary, our study demonstrates that human T H 1/17 cells and IL-10 − T H 17 clones display significant similarities to mouse pathogenic T H 17 cells in their transcriptomic patterns. The elevated expression of pro-inflammatory cytokines and chemokines in human IFN-γ-secreting T H 17 cells and the similarity in gene expression profiles between human IFN-γ-secreting T H 17 cells and mouse pathogenic T H 17 cells indicates a higher pro-inflammatory capacity of human T H 1/17 cells and additionally provides transcriptional evidence to support the role of human T H 1/17 in the pathogenesis of human autoimmune diseases. The differential molecular signature of human IFN-γ-secreting T H 17 cells that we identified provides a new tool that can be utilized to assess T H 17 cells both under physiologic conditions and in association with disease. Reagents EasySep human CD4 + T-cell enrichment kit (catalog number 19052) for CD4 + T-cell isolation was purchased from StemCell Technologies. FITC-conjugated anti-human IFN-γ (clone, B27; 1:100), Alexa 647-conjugated anti-human IL-17A (clone, N49-653; 1:20), PE-conjugated anti-human IL-10 (clone, JES3-19F; 1:660), and their corresponding isotype control antibodies for intracellular cytokine staining assay were purchased from BD Biosciences. IFN-γ cytokine secretion detection kit (APC) (catalog number 130-090-762) and IL-17 cytokine secretion detection kit (PE) (catalog number 130-094-537) were purchased from Miltenyi Biotec. nCounter CodeSet HuT H 17 was custom designed and manufactured by nanoString Technologies. Fluorescence-conjugated antibodies for cell surface staining for flow cytometry were purchased from Biolegend. RNAqeous micro total RNA isolation kit (catalog number AM1931), SuperScript VILO master mix (catalog number 11755050), TaqMan preAmp master mix (catalog number 4391128), TaqMan fast universal PCR master mix (2x) (catalog number 4352042), and qPCR primers (Supplementary Data 8 ) were purchased from ThermoFisher Scientific. Human subjects Blood samples for T H 17 cloning from healthy donors were obtained from the Swiss Blood Donation Center of Basel and Lugano. Informed, written consent was obtained from all donors. All uses of human material were approved by the Federal Office of Public Health (authorization no. A000197/2 to F.S.). Blood samples from MS patients and healthy controls were obtained from the Partners MS Center at Brigham and Women’s Hospital under IRB Protocol 2001P001431 and 2014P000124. Informed, written consent was obtained from all donors. MS patients were untreated for a minimum of 6 months before sampling. Disease activity was identified as a gadolinium-enhancing lesion on MRI or disease relapse within 6 months of sampling. Age- and sex-matched healthy donors did not have history of autoimmune diseases or malignancies and no acute or chronic infections. The samples from healthy donors for nCounter gene expression analysis were fresh blood samples. The MS samples and age- and sex-matched healthy control samples were frozen peripheral blood mononuclear cells (PBMCs). Intracellular cytokine staining For intracellular cytokine staining for PBMC or CD4 + T cells, assays were carried out with staining buffers and antibodies from BD Biosciences. Briefly, cells were seeded into a 96-well plate (up to 1 × 10 6 cell per well) and stimulated with PMA (100 ng/ml) and ionomycin (1 μg/ml) in the presence of GolgiStop for 4 h. After stimulation, cells were fixed with BD Cytofix fixation buffer and washed with BD Perm/Wash buffer. Cells in each well were equally divided into two wells, with one for intracellular cytokine staining and the other for isotype control staining. The following fluorophore-conjugated antibodies from BD Biosciences were used for staining analysis or as isotype controls: anti-CD4-pacific blue (clone: RPA-T4; 1:330), anti-IL-17A-Alexa647 (clone: N49-653; 1:20), anti-IFN-γ-FITC (clone: B27: 1:100), anti-IL-10-PE (clone: JES3-19F: 1:660), mouse IgG1-Alexa647 (clone: MOPC-21; 1:40), mouse IgG1-FITC (clone: MOPC-21; 1:100), and rat IgG2a-PE (clone: R35-95: 1:660). Stained cells were analyzed with a BD LSR II cytometer. Cytokine secretion in CD4 + lymphocytes was accessed with FlowJo. Isolation of viable T H subsets from human PBMC PBMC isolated with Ficoll-Pague PLUS (GE Healthcare) gradient centrifugation from the peripheral blood of healthy donors. Total CD4 + T cells were purified with the EasySep human CD4 + T-cell enrichment kit (StemCell Technologies). CD4 + T cells seeded in a 96-well plate (1 × 10 6 cells/well) were stimulated with PMA (30 ng/ml) and ionomycin (1 μg/ml) for 3–4 h (3 h for fresh blood samples and 4 h for frozen PBMC samples). Viable T H 1/17, T H 17, T H 1, and DN cells were sorted with a FACSAria (BD Biosciences) after being stained with IFN-γ and IL-17 cytokine secretion detection kits (Miltenyi Biotec) and fluorescence-conjugated anti-CD3 and anti-CD4 antibodies following the manufacturer’s suggested protocol. Isolation of human IL-10 − and IL-10 + T H 17 clones PBMC were isolated by Ficoll-Paque PLUS (GE Healthcare) separation. CD4 + T cells were isolated from PBMC by positive selection using CD4 magnetic microbeads (Miltenyi Biotec). CCR6 + CCR4 + CXCR3 – CD45RA – CD25 – CD8 – CD14 – CD19 – CD56 – (enriched in T H 17 cells) memory CD4 T cells were sorted with a FACSAria (BD Biosciences) and seeded at 0.6 cells per well in a 384 well plate. The following antibodies were used for FACS-based sorting: anti-CD45RA-Qdot655 (Life Technologies; clone: MEM-56; 1:1000); anti-CCR7-BV421 (Biolegend; clone: G043H7; 1:80); anti-CCR6-PE (BD Biosciences; clone: 11A9; 1:80) or anti-CCR6-BV605 (Biolegend; clone: G034E3; 1:60); anti-CCR4-PECy7 (BD Biosciences; clone: 1G1; 1:100); anti-CXCR3-PE-Cy5 or anti-CXCR3-APC (BD Biosciences; clone: 1C6; 1:20); anti-CD8-FITC or anti-CD8-PE-Cy5 (Beckman Coulter; clone: B9.11; 1:25); anti-CD25-FITC or anti-CD25-PE-Cy5 (Beckman Coulter; clone: B1.49.9; 1:25); anti-CD14-FITC or anti-CD14-PE-Cy5 (Beckman Coulter; clone: RMO52; 1:25); anti-CD19-FITC (BD Biosciences, clone: HIB19), or anti-CD19-PE-Cy5 (Beckman Coulter; clone: J3-119; 1:25); CD56-PE-Cy5 (Beckman Coulter; clone: N901; 1:25). CD4 T-cell clones were established in the presence of irradiated (45 Gy) allogeneic PBMC (25,000 cells per well) and phytohaemagglutinin (PHA-L) (1 μg/ml) in medium supplemented with IL-2 (500 U/ml). A small portion of cells of each CD4 + T-cell clone was used for intracellular cytokine staining assay for IL-17A (anti-IL-17A-eF660; eBioscience, catalog number 50-7179-42 clone: eBio64DEC17; 1:200), IL-10 (anti-IL-10-PE; BD Biosciences, catalog number 559330; clone: JES3-19F1; 1:20), and IFN-γ (anti-IFN-γ-FITC; BD Biosciences, catalog number 554700; clone: B27; 1:800) production. IL-10 – and IL-10 + T H 17 clones were selected for further analysis. Regular quantitative real-time PCR To measure gene expression in T H 17 clones with qPCR, IL-10 – and IL-10 + T H 17 clones from an individual donor were pooled. They were stimulated or not with plate-bound anti-CD3 (clone TR66, 5 μg/ml) and anti-CD28 (clone CD28.2, 1 μg/ml) (αCD3/CD28) for 4 h, or stimulated with αCD3/CD28 for 5 days followed with or without a second αCD3/CD28 treatment for 4 h. Pooled T H 17 clone cells were subjected to RNA isolation. Total RNA was extracted with the E.Z.N.A. Total RNA kit I (Omega Bio-tek, product number R6834). qPCR analysis was run and analyzed with the ViiA 7 Real-Time PCR System (Life Technologies). Quantitative comparison between IL-10 – and IL-10 + T H 17 clones was calculated using comparative Δ C T . Gene expression was normalized to the expression of β2 m. Low-input quantitative real-time PCR To measure gene expression in T H 1/17, T H 17, T H 1, and DN cells sorted from frozen PBMC with qPCR, total RNA was isolated and digested with DNase I with the RNAqeous micro total RNA isolation kit. cDNA was synthesized with the SuperScript VILO master mix and pre-amplified for 14 cycles with the TaqMan preAmp master mix following the manufacture’s instruction. qPCR analysis was run and analyzed with the ViiA 7 Real-Time PCR System (Life Technologies) using the TaqMan fast universal PCR master mix (2x) and qPCR primers purchased from ThermoFisher Scientific. The comparative threshold cycle method and an internal control ( β2m ) were used for normalization of the target genes. Relative expression was calculated as: Δ C T = C Tgene of interest – C Tβ2m ; ΔΔ C T = Δ C T cell subset of interest – mean of Δ C T DN of healthy control ; the relative change of gene expression between the expression level of sample of interest and the mean expression level of all DN samples in healthy controls was given by this formula: (2 –ΔΔ C T ) × 10. All qPCR reactions were performed in duplicate. nCounter analysis of mRNA expression We designed a nanoString CodeSet HuT H 17 that constitutes a 418-gene expression detection panel specific for human T-cell activation and differentiation (Supplementary Data 1 ). 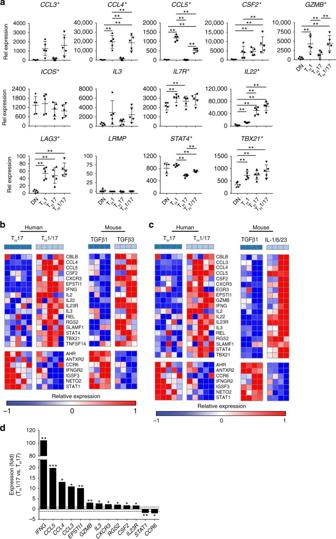Fig. 2 Gene expression comparison between human TH1/17 vs. TH17 cells and mouse pathogenic vs. non-pathogenic TH17 cells.aThe expression of previously reported murine and human TH17 signature genes in purified ex vivo TH1 cells. The mRNA gene expression levels in TH1/17, TH17, TH1, and DN cells were measured as described in Fig.1. *p< 0.05, repeated measures one-way ANOVA; **p< 0.05, pairwised group comparison with Tukey’s multiple comparison test (mean ± s.d.,n= 5).b,cGene set enrichment analysis comparing human TH1/17 vs. TH17 cells with mouse pathogenic vs. non-pathogenic TH17 cells.bHeatmap of upregulated (upper panels) and downregulated (lower panels) “leading edge” genes of comparison Scenario 1: human TH1/17 vs. TH17 cells vs. mouse TGF-β3 plus IL-6-induced TH17 cells vs. TGF-β1 plus IL-6-induced TH17 cells (Kolmogorov–Smirnov testp< 0.0001; FDRq< 0.0001 for upregulated genes; Kolmogorov–Smirnov testp= 0.0007; FDRq= 0.001 for downregulated genes).cHeatmap of upregulated (upper panels) and downregulated (lower panels) “leading edge” genes of comparison Scenario 2: human TH1/17 vs. TH17 cells vs. mouse IL-1, IL-23 plus IL-6-induced TH17 cells vs. TGF-β1 plus IL-6-induced TH17 cells (Kolmogorov–Smirnov testp< 0.0001; FDRq< 0.0001 for upregulated genes; Kolmogorov–Smirnov testp= 0.004; FDRq= 0.004 for downregulated genes). Each column represents one donor in human(n= 5) or one sample in murine (n= 4).dThe robust predicted pathogenic signature (PreP-Signature) of human TH1/17 cells. Signature genes are those identified as differentially expressed between human TH1/17 and TH17 cells that are identified as enriched “leading edge” genes when assessing these human genes in the mouse profiles inb,cand that are additionally curated for robustness based on supervised absolute fold change >1.5. Two tailed, paired Student’sttestp-value < 0.05. *p< 0.05, **p< 0.05, ***p< 0.0005,n= 5 Cell lysates were prepared from sorted T H 1/17, T H 17, T H 1, and DN cells with the RLT-Plus buffer of the RNeasy Plus Mini Kit (Qiagen, catalog number 74134) and gene expression levels were generated using the CodeSet HuT H 17 according to the protocol provided by the manufacturer (NanoString Technologies). For gene expression in IL-10 − and IL-10 + T H 17 clones, total RNA was used for nCounter analysis following the manufacturer’s suggested protocol (NanoString Technologies). Data analysis nCounter gene expression data were normalized for code count using the geometric mean, for background using the mean, and for sample content using the geometric mean of housekeeping genes (isolated human CD4 + T-cell subsets: B2M , RPL3 , and beta actin; human T H 17 clones: B2M , GAPDH , and beta actin) with the R 3.2.0. NanoStringNorm package. 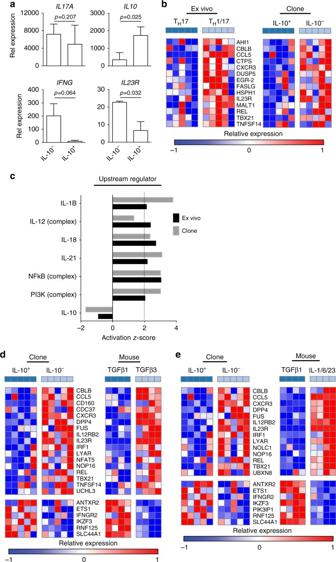Fig. 3 Gene expression comparison between human TH1/17 vs. TH17 cells and IL-10–vs. IL-10+TH17 clones.aQuantitative RT-PCR analysis of gene expression in human IL-10–and IL-10+TH17 clones isolated from healthy donors (two tailed, paired Student’sttest, mean ± s.d.,n= 3). ForIFNG,IL17A, andIL23R, resting TH17 clones were stimulated with anti-CD3 and anti-CD28 for 4 h before RNA extraction. ForIL10, resting TH17 clones were stimulated with anti-CD3 and anti-CD28 for 5 days, then cells were re-stimulated with anti-CD3 and anti-CD28 for 4 h before RNA extraction.bHypergeometric enrichment test between human TH1/17 vs. TH17 cells and IL-10–vs. IL-10+TH17 clones. Genes differentially expressed between human TH1/17 and TH17 cells (Supplementary Data3) were analyzed for enrichment in those of human IL-10–vs. IL-10+TH17 clones (Supplementary Data5). Heatmap shows the overlapping genes (one-sided Fisher’s exact testp< 0.0001, FDRq= 0.0001). Each column represents one donor (n= 5).cPredicted upstream regulators for TH1/17 and IL-10–TH17 clone differentiation. The differentially expressed genes with corresponding fold changes andp-values from the TH1/17 vs. TH17 comparison (Supplementary Data3) and IL-10–vs. IL-10+TH17 clone comparison (Supplementary Data5) were analyzed using the IPA upstream regulator analysis. Ex vivo, TH1/17 vs. TH17 comparison; Clone, IL-10–vs. IL-10+TH17 clone comparison.d,eGene set enrichment analysis comparing human IL-10–vs. IL-10+TH17 clones with mouse pathogenic vs. non-pathogenic TH17 cells.dHeatmap of upregulated (upper panels) and downregulated (lower panels) “leading edge” genes of comparison Scenario 1: human IL-10–vs. IL-10+TH17 clones vs. mouse TGF-β3 plus IL-6-induced TH17 cells vs. TGF-β1 plus IL-6-induced TH17 cells (Kolmogorov–Smirnov testp= 0.004; FDRq= 0.005 for upregulated genes; Kolmogorov–Smirnov testp= 0.004; FDRq= 0.003 for downregulated genes).eHeatmap of upregulated (upper panels) and downregulated (lower panels) ‘‘leading edge” genes of comparison Scenario 2: human IL-10–vs. IL-10+TH17 clones vs. mouse IL-1, IL-23 plus IL-6-induced TH17 cells vs. TGF-β1 plus IL-6-induced TH17 cells (Kolmogorov–Smirnov testp= 0.005; FDRq= 0.010 for upregulated genes; Kolmogorov–Smirnov testp= 0.016; FDRq= 0.009 for downregulated genes). Each column represents one donor in human (n= 5) or one sample in murine (n= 4) 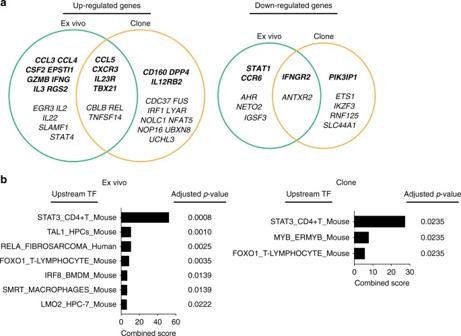Fig. 4 Predicting STAT3 as upstream transcription factor by the PreP-Signatures of TH17 cells.aVenn diagram representations of signature genes upregulated (left) and downregulated (right) in human TH1/17 cells and IL-10–TH17 clones. Complete PreP-Signatures from GSEA comparison Scenarios I and II were merged for ex vivo cells (Fig.2b, c) and TH17 clones (Fig.3d, e), respectively. Genes with supervised absolute fold change >1.5 in either ex vivo cells or TH17 clones were shown in italic bold letters. Ex vivo, differentially expressed “leading edge” genes from TH1/17 vs. TH17 GSEA comparisons presented in green circles; Clone, differentially expressed “leading edge” genes from IL-10–vs. IL-10+TH17 clone GSEA comparisons presented in yellow circles.bPredicted upstream transcription factors for TH1/17 and IL-10–TH17 clone differentiation. The molecular signatures of TH1/17 cells and IL-10–TH17 clones inawere analyzed using the Enrichr ChEA2016 analysis and the predicted transcription factors with Benjamini–Hochberg adjustedp-value <0.05 were shown. TF transcription factor Mouse gene expression data were downloaded from GEO (GSE39820) and normalized using RMA [62] and ComBat [63] in GenePattern ( http://www.broadinstitute.org/cancer/software/genepattern/ ) as previously published [12] . Genes for which multiple probes were measured on the mouse microarray were collapsed to unique genes by selecting the probe with the highest average expression across all samples. Hierarchical clustering of the human samples and of the pairwise Pearson linear correlations were done based on the 362 genes that varied across the population in an unbiased manner (unsupervised expression difference (Δ = maximum expression value – minimum expression value)≥5, defined as the difference between maximum and minimum relative gene expression values across the population without considering the subset classes) using Pearson linear correlation and average linkage in GENE-E. PCA of the isolated human CD4 + T-cell subsets was done in R (prcomp) based on the same 362 genes. We selected differentially expressed genes between T H 1/17 and T H 17 cells using the two tailed, paired Student’s t test followed by supervised filtering for expression differences between mean T H 1/17 and mean T H 17 (Δ = MEAN TH1/17 −MEAN TH17 )>20 for robustness. The same approach was used to select differentially expressed genes between IL-10 − and IL-10 + T H 17 clones. GSEA was done in GenePattern using default settings (weighted scoring scheme, Signal2Noise metric, 1000 permutations) [34] , [64] , [65] to test the enrichment of human signatures in the mouse expression profiles. Gene set overlap statistic analysis was done using the hypergeometric test in R (phyper, with N equal to the number of genes measured on the NanoString CodeSet). Storey’s q -value is used to control the FDR. Visualization of the gene expression heatmaps was done in GENE-E [ http://www.broadinstitute.org/cancer/software/GENE-E/ ]. Il23r was not included in our microarray chip for mouse T H 17 cell analysis, but we found upregulation of Il23r in murine pathogenic T H 17 cells by qPCR [12] . Thus, we included Il23r in the murine gene expression profiles. The IPA upstream regulator analysis was performed for the differentially expressed genes (using corresponding fold changes and p -values) to identify key upstream regulatory molecules. Upstream regulators with z -scores >2 and z -scores <−2 represent activator and inhibitor mechanisms, respectively. The Enrichr ChEA2016 database and analytic tools were used to predict key upstream transcription factors [36] , [37] . Statistical analysis Statistical analysis was performed with Prism 7 (GraphPad Software), R statistical software (version 3.2.0), and Excel version 14.4.7. One-way analysis of variance with Tukey’s multiple comparison test was performed to compare the differential gene expression among T H subsets within HCs or MS patients when more than two cell subsets were included, while two tailed, paired Student’s t test was performed when only two cell subsets were included. Welch’s t test (unpaired t test with Welch’s correction) was performed to compare the differential gene expression between healthy controls and MS patients on a specific T H subset. Two sided p -values of <0.05 were considered statistically significant. Code availability Computer code used to generate results is available from the corresponding author upon request. Data availability The authors declare that the main data supporting the findings of this study are available within the article and its Supplementary Information files. 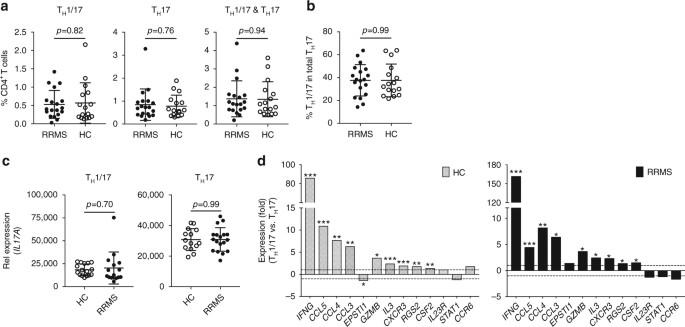Fig. 5 Frequency of TH17 subsets and differential expression of PreP-Signature genes in TH1/17 vs. TH17 cells in MS. Peripheral CD4+T cells isolated from the PBMC of untreated RRMS patients (n= 19) and age- and sex-matched healthy controls (HC) (n= 16) were stimulated, stained, and sorted for TH1/17, TH17, TH1, and DN cells as described in Fig.2b. RNA isolated from sorted cell subsets was subjected to low-input qPCR analysis.aFrequencies of TH1/17, TH17, and total TH17 cells in total peripheral CD4+T cells (Welch’sttest,p-values, mean ± s.d.).bFrequency of TH1/17 in total TH17 cells (Welch’sttest, mean ± s.d.).c,dqPCR analysis of gene expression in isolated CD4+T-cell subsets.cComparison ofIL17Aexpression between HC and patients in TH1/17 or TH17 cells (Welch’sttest, mean ± s.d.).dDifferential expression of PreP-Signature genes between TH1/17 vs. TH17 cells in HC and MS patients. Two tailed, paired Student’sttest, *p< 0.05, **p< 0.001, ***p< 0.0001 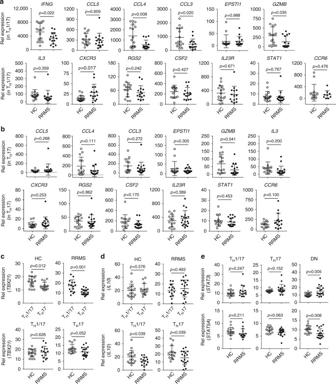Fig. 6 Expression of PreP-signature genes of human pro-inflammatory TH17 cells in RRMS. RNA isolated from TH1/17, TH17, and DN cells (Fig.5) was subjected to qPCR analysis. Comparison of PreP-Signature gene expression between HC and patients with RRMS inaTH1/17 cells andbTH17 cells. (Welch’sttest, mean ± s.d.). Comparison ofcTBX21anddIL10expression between HC and patients with RRMS in TH1/17 and TH17 cells.eComparison ofSTAT3(upper panel) andSTAT5A(lower panel) expression between HC and patients with RRMS in TH1/17, TH17, and DN cells. Welch’sttestp-values were shown (mean ± s.d.) 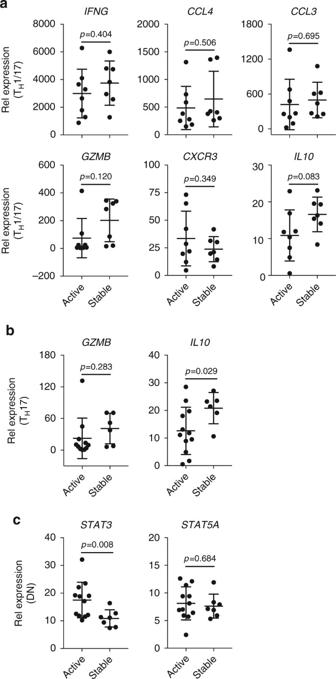Fig. 7 Correlation ofIL10andSTAT3expression with disease activity in MS. The mRNA levels of signature genes with altered expression in MS (Fig.6) were compared between active and stable patients. Signature gene expression inaTH1/17 (active,n= 8; stable,n= 7),bTH17 (active,n= 12; stable,n= 6), andcDN cells (active,n= 12; stable,n= 7) (Welch’sttest, mean ± s.d.) Gene expression data that support the findings of this study have been deposited in the Gene Expression Omnibus with the accession code (GSE104024). (All other relevant data are available from the corresponding author upon reasonable request.